Biomimetic layer-by-layer assembly of artificial nacre Nacre is a technologically remarkable organic–inorganic composite biomaterial. It consists of an ordered multilayer structure of crystalline calcium carbonate platelets separated by porous organic layers. This microstructure exhibits both optical iridescence and mechanical toughness, which transcend those of its constituent components. Replication of nacre is essential for understanding this complex biomineral, and paves the way for tough coatings fabricated from cheap abundant materials. Fabricating a calcitic nacre imitation with biologically similar optical and mechanical properties will likely require following all steps taken in biogenic nacre synthesis. Here we present a route to artificial nacre that mimics the natural layer-by-layer approach to fabricate a hierarchical crystalline multilayer material. Its structure–function relationship was confirmed by nacre-like mechanical properties and striking optical iridescence. Our biomimetic route uses the interplay of polymer-mediated mineral growth, combined with layer-by-layer deposition of porous organic films. This is the first successful attempt to replicate nacre, using CaCO 3 . Nacre's biogenic synthesis process entails a symphony of mineral and organic species, which finely control each others' deposition [1] , [2] . Nacre forms extracellularly in the isolated space between the shell and the epithelium mantle cells. These cells secrete porous hydrophobic chitin sheets that are covered by acidic silk proteins, which form a boundary between mineral layers. Mineralization then proceeds by the deposition of a chemically stabilized CaCO 3 amorphous (ACC) precursor phase [3] , [4] onto the chitin sheets, where it coalesces to form an ACC film. The repeated deposition of chitin and ACC followed by CaCO 3 crystallization leads to a lamellar stacks of CaCO 3 tablets separated by organic layers. The porosity of the chitin layers is an important structural feature, allowing mineral interconnects, which are responsible for crystal continuity between the platelets, improving the mechanical properties of the stack [5] . The characteristic nacre structure in Fig. 1a–c consists of 250–500 nm thick aragonite tablets, separated by 30–90 nm thick organic layers [2] , seen in Fig. 1b . Each tablet is part of a single crystal, and the crystallinity extends though tablet stacks, mediated by holes [1] (mineral interconnects) in the organic layers in Fig. 1c . The stack periodicity give rise to the hallmark iridescence of nacre shown for a shell of Haliotis tuberculata in Fig. 1a . 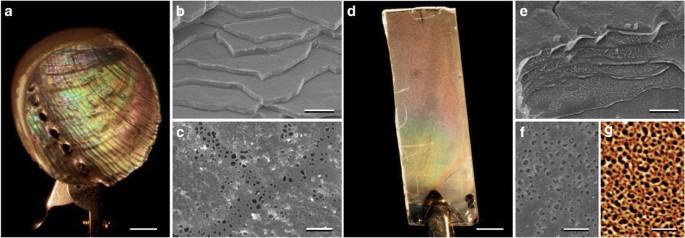Figure 1: Comparison of biogenic and artificial nacre. (a) Photograph showing nacre's bright iridescence (scale bar, 5 mm). (b) Fractured surface SEM image of a stack of mineral tablets (scale bar, 2 μm). (c) Organic inter-crystalline, film which allows for vertical crystal continuity between tablets (scale bar, 500 nm). (d) Artificial nacre, exhibiting a similar coloration as ina(scale bar, 5 mm). (e) SEM image of a fractured surface showing seven aligned CaCO3tablets separated by organic films. The surface graininess is comparable to natural nacre (scale bar, 1 μm). (f) SEM image of a PVP film on calcite showing the a similar pore distribution as in (c) (scale bar, 300 nm). (g) atomic force microscope (AFM) height image of the porous film (scale bar, 300 nm). Figure 1: Comparison of biogenic and artificial nacre. ( a ) Photograph showing nacre's bright iridescence (scale bar, 5 mm). ( b ) Fractured surface SEM image of a stack of mineral tablets (scale bar, 2 μm). ( c ) Organic inter-crystalline, film which allows for vertical crystal continuity between tablets (scale bar, 500 nm). ( d ) Artificial nacre, exhibiting a similar coloration as in a (scale bar, 5 mm). ( e ) SEM image of a fractured surface showing seven aligned CaCO 3 tablets separated by organic films. The surface graininess is comparable to natural nacre (scale bar, 1 μm). ( f ) SEM image of a PVP film on calcite showing the a similar pore distribution as in ( c ) (scale bar, 300 nm). ( g ) atomic force microscope (AFM) height image of the porous film (scale bar, 300 nm). Full size image Although organic/inorganic composites are common in nature and technology, nacre, as well as sea-urchin spines and skeletons, has intrigued scientists because these organisms are able to mould large single-crystal shapes and create materials that fulfil specific functions for the organisms [6] , [7] , [8] . Replicating nacre is interesting as it sheds light on the biological processes at work in growing this biomineral, and it equips us to fabricate novel tough coatings using low cost materials in ambient conditions. Although other studies have identified many complex biochemical pathways that lead to nacre's biomineral growth [1] , [4] , [9] , here we propose a minimum of five essential stages, which are necessary to successfully mimic nacre: (1) Stabilization of ACC in solution, (2) Specific aggregation and continuous film formation on organic surfaces, (3) Deposition of a porous, suitably functionalized thin organic film on a previously formed mineral layer, (4) Crystallization of the formed ACC layers to aragonite or calcite and (5) Cyclical iteration of steps 1–4. Previous attempts at mimicking nacre only aimed at some of these five steps. In particular, they lacked mineral continuity across the porous organics, and thus failed to achieve nacre's characteristic microstructure [10] , [11] , [12] . Nacre has previously been retro-synthesized by recrystallizing the decalcified insoluble organic matrix of an abalone shell [13] . The organic–inorganic hybrid principle of nacre has been followed in the creation of several non-calcareous systems [14] , [15] , [16] , [17] , [18] , [19] . Here, we report a route to a nacre-like CaCO 3 multilayer that includes all five steps outlined above, resulting in a stack of crystalline calcite layers, interconnected though porous organic films. Both the growth strategy and final material bear close resemblance to biogenic nacre. Fabrication Our experimental procedure is illustrated in Fig. 2 . Initially, layer-by-layer deposition of two polyelectrolytes was used to form a continuous organic thin film [20] , [21] by cyclicly immersing a glass substrate into poly (acrylic acid) (PAA) and poly (4-vinyl pyridine) (PVP) solutions until the desired film thickness was obtained ( Fig. 1a ). The film is then immersed into a pH 10 solution, dissolving the PAA and inducing a positive charge on the substrate and in the PVP. The resulting repulsive interaction leads to nanopore formation by PVP dewetting, which is quenched and stabilized by UV cross-linking [22] . A final immersion into PAA solution functionalizes the PVP surface with COO − groups to promote mineral deposition ( Fig. 2b ). 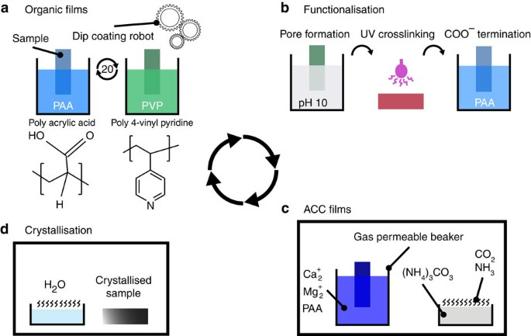Figure 2: Scheme of artificial nacre synthesis. (a) A continuous PAA/PVP film was formed by sequentially immersing a glass slide into PAA and PVP solutions for 1 min each. (b) Transformation of the layer into a porous film: Immersion in a basic solution dissolves PAA and induces pores by dewetting. Stabilization by UV cross-linking. Surface functionalization by PAA immersion. (c) Mineral film formation in close contact with gas permeable beaker wall. Polymer-induced liquid precursor (PILP) droplets form by CO2diffusion, stabilized by included PAA and Mg to form a modified calcite (calorg) film. (d) Crystallization of the most recently deposited calorglayer. Each full cycle produces a single organic/mineral bilayer, which is repeated to create a stack. Figure 2: Scheme of artificial nacre synthesis. ( a ) A continuous PAA/PVP film was formed by sequentially immersing a glass slide into PAA and PVP solutions for 1 min each. ( b ) Transformation of the layer into a porous film: Immersion in a basic solution dissolves PAA and induces pores by dewetting. Stabilization by UV cross-linking. Surface functionalization by PAA immersion. ( c ) Mineral film formation in close contact with gas permeable beaker wall. Polymer-induced liquid precursor (PILP) droplets form by CO 2 diffusion, stabilized by included PAA and Mg to form a modified calcite (cal org ) film. ( d ) Crystallization of the most recently deposited cal org layer. Each full cycle produces a single organic/mineral bilayer, which is repeated to create a stack. Full size image Mineral growth in Fig. 2c is based on the biological strategy using ACC [23] , [24] , [25] , [26] . Using the ammonium carbonate diffusion technique with a PAA-containing 1:5 Ca 2+ :Mg 2+ solution (Mg 2+ and PAA suppress calcite rhombohdra formation) [27] yields stable polymer-induced liquid precursor droplets, which wet the carboxyl terminated substrate and coalesce into a ACC film, rich in Mg and PAA (cal org ) [28] , [29] . A key advance in extending this mineral deposition technique to create large (10 cm 2 ) high quality films is the confinement of the reaction volume by a gas permeable membrane, providing uniform distribution of CO 2 in the solution. The ACC is then crystallized by exposure to high humidity, allowing for a dissolution–recrystallization transformation [30] ( Fig. 2d ). The propagation of crystallization occurs through the organic pores, connecting the mineral layers. The fabrication of an organic/cal org bilayer (an entire cycle of steps a–d) can be achieved in 5 h, making it viable to grow many multilayers via repetition. Microstructure The resulting material is highly comparable to biogenic nacre (compare Fig. 1a–c with d–g ) both in its morphology and growth route. In particular, a comparison of the scanning electron microscopy (SEM) image of fractured surfaces of biogenic ( Fig. 1b ) and artificial ( Fig. 1e ) nacre reveals very similar multilayers of 400-nm thick cal org tablets with a nano-granular texture that is characteristic of nacre. A key advantage of our route to artificial nacre is the fabrication of the porous organic inter-crystalline layers, which are comparable to those in natural nacre ( Fig. 1c,f,g , Supplementary Table S1 and Supplementary Fig. S2 ). These pores allow bridges between the mineral films to form, providing vertical crystalline mineral continuity, which enhances nacre's mechanical stability [5] , [9] . Without these interconnects the layered structure is unstable during growth and delaminates. This is readily demonstrated by modifying step b in Fig. 2 , so that no pores are formed in the organic layers. This leads to highly unstable stacks of delaminating layers ( Supplementary Fig. S3 ). Earlier approaches were also plagued by the delamination of non-connected layers caused by the stresses arising from the dehydration of ACC [10] , [11] , [12] . The pores allow the propagation of crystallization across the organic layers, which promotes biomimetic crystal sizes that span a number of layers. 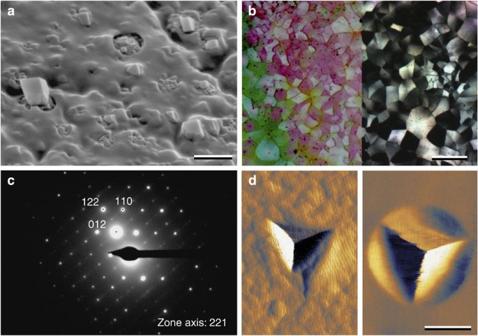Figure 3: Characterization of artificial nacre crystallinity. (a) SEM image showing early-stage crystallization through single PVP pores in a trilayer of calorg/organic/calorg(scale bar, 500 nm). (b) Optical micrograph showing 5–35 μm birefringent crystalline domains (right: though crossed polarisers) (scale bar, 25 μm). (c) TEM-SAED of a single tablet evidencing calcite single crystallinity. (d) Cube corner indentation (imaged by atomic force microscopy, AFM) caused crack formation in a calorgfilm (left) and plastic deformation in a seven-layer artificial nacre sample (right), similar to biogenic nacre (Supplementary Fig. S9) (scale bar, 1 μm). Figure 3a confirms the role of the pores in crystal propagation. Quenching the crystallization of the amorphous top layer after only 10 min followed by dissolution of the remaining amorphous material reveals facetted seed crystallization in the pores (also Supplementary Figs S4 and S5 ). Facets are suppressed while the mineral is in contact with a soft organic material, but crystallinity is nevertheless propagated through the pores, in agreement with previous studies [23] , [24] . Figure 3: Characterization of artificial nacre crystallinity. ( a ) SEM image showing early-stage crystallization through single PVP pores in a trilayer of cal org /organic/cal org (scale bar, 500 nm). ( b ) Optical micrograph showing 5–35 μm birefringent crystalline domains (right: though crossed polarisers) (scale bar, 25 μm). ( c ) TEM-SAED of a single tablet evidencing calcite single crystallinity. ( d ) Cube corner indentation (imaged by atomic force microscopy, AFM) caused crack formation in a cal org film (left) and plastic deformation in a seven-layer artificial nacre sample (right), similar to biogenic nacre ( Supplementary Fig. S9 ) (scale bar, 1 μm). Full size image Although SEM and atomic force microscope images of the cal org tablets do not resolve any crystal grain boundaries, optical microscopy between cross-polarisers reveals a polycrystalline structure with grain sizes in the 5–35 μm range ( Fig. 3b ). This is much larger than any other length scale (tablet thickness, pore-size and distance and so on) in the material. The single-crystal nature of the large domains was confirmed by transmission electron microscopy (TEM)-selected area electron diffraction (SAED) of individual tablets ( Figs 1c ,5). The similarity of crystal domain size in Fig. 1b to natural nacre [31] is remarkable, given the close pore spacing of the organic interlayers. The step-by step nature of our approach allows to elucidate the origin of the crystal domain size. The investigation of only on single layer shows a similar crystal morphology as the stack ( Supplementary Fig. S6 ). The crystal domain size is therefore determined by the nucleation density of the first layer, which can be controlled by the relative Mg content [29] . Despite the high pore density and 10 nm pore size, the lateral crystal morphology is preserved in successive layers. To this end it is necessary that the crystal growth through the pores has the same spatial symmetry, leading to a nanogranular morphology of grains that have the same crystallographic orientation and therefore give rise to the clear diffractogram of Fig. 3c . Mineral continuity across the organic sheets is therefore important to maintain the co-orientation of all tablets in the columnar stack [31] , their crystal structure and the mechanical cohesion of the layered structure. Mechanical properties The similar morphology of natural and artificial nacre is evidenced by comparable mechanical properties. First, mean plain strain moduli of 69, 38, 176, 86 and 10 GPa for natural and artificial nacre, aragonite, cal org and PVP, respectively, were measured ( Supplementary Fig. S7 ). The smaller elastic modulus of artificial nacre, compared with natural nacre, is a direct consequence of PAA and Mg inclusion within cal org , seen in Supplementary Fig. S8 . The modulus of both nacre types is well described by 1/ E nacre = φ 1 / E 1 + φ 2 / E 2 , where φ i is the volume fraction of the (1) inorganic and (2) organic phases. The very similar morphologies therefore give rise to identical ratios of moduli of natural/artificial nacre to aragonite/cal org , respectively. More important than the stiffness characteristics mimicking natural nacre, the fracture toughness was qualitatively probed by cube-corner indentation ( Fig. 3d ). This showed plastic deformation in artificial nacre, under loads that cracked solid cal org , demonstrating the toughening of the alternating cal org -PVP stack. This result is analogous to the comparison of toughening of aragonite in natural nacre ( Supplementary Fig. S8 ). Optical properties The similarities in iridescence between biological and artificial nacre ( Fig. 1a,d ) were spectroscopically investigated. 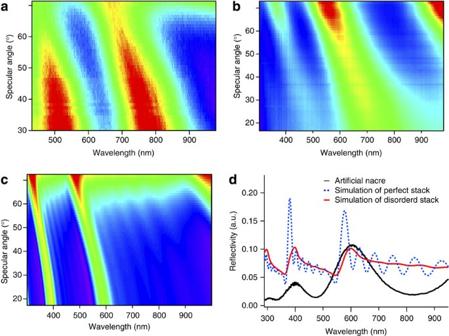Figure 4: Optical characterization. Reflectivity as a function of wavelength and reflection angle showing (a) biogenic and (b) artificial nacre containing seven bilayers (bilayer=calorg/organic). The wavelength-dependent angles of maximal intensity (red) extending diagonally across the images result from multilayer interference. (c) Simulation of a seven-bilayer stack of artificial nacre. The mineral thickness was averaged over ±15 nm to factor in disorder. (d) The reflection profile from (b) at an angle of 35° is compared with a calculated spectrum of a perfect CaCO3/PVP multilayer and a spectrum cut from the disordered simulation in (c). Figure 4a,b show the specularly reflected signal as a function of incident angle and wavelength for the two types of nacre. Both spectra have the same salient features: the two prominent reflection bands that diagonally span the spectra correspond to second- and third-order interference, which is characteristic of multiayer stacks. The similar location and width of these spectral features lies at the origin of the similar macroscopic optical appearance of Fig. 1a,c . The difference between the two stems from the variation of the intensity of the interference bands with angle, which arises from the increased scattering in biogenic nacre. The spectral response of the artificial nacre was compared with a simulated seven-bilayer system in Fig. 4c,d . A perfect stack has very narrow interference peaks and minor oscillations stemming from its finite size. Including irregularities by introducing layer thickness variations of ±15 nm gives rise to a simulated spectrum, which qualitatively approaches the measured specular reflection of artificial nacre, seen in Fig. 4c,d . The broader interference bands in Fig. 4a,b also arise from scattering, which was not included in the simulation. Figure 4: Optical characterization. Reflectivity as a function of wavelength and reflection angle showing ( a ) biogenic and ( b ) artificial nacre containing seven bilayers (bilayer=cal org /organic). The wavelength-dependent angles of maximal intensity (red) extending diagonally across the images result from multilayer interference. ( c ) Simulation of a seven-bilayer stack of artificial nacre. The mineral thickness was averaged over ±15 nm to factor in disorder. ( d ) The reflection profile from ( b ) at an angle of 35° is compared with a calculated spectrum of a perfect CaCO 3 /PVP multilayer and a spectrum cut from the disordered simulation in ( c ). Full size image Single crystallinity across organic layers Figure 1 shows evidence of crystal continuity across one organic layer. The selected area diffraction in Fig. 1b was performed over a 1-μm-wide area, including comparable areas on both sides of the organic layer (delimited by dashed lines in Fig. 1a ). The bright indexed spots indicate a single crystalline material, although some weak background spots can be seen. This might be caused by a small minority of alternatively ordered crystals, although the signal could simply arise from the ion-milling process. It was not possible to find a cross-section that included a calcite bridge across an organic pore. We are, however, confident that the interconnecting mineral bridges are the source of this crystalline continuity, because in their absence there is no mechanism for crystalline orientation to propagate across the 30 nm thick amorphous organic layers. The proliferation of crystallinity across a stack of tablets requires physical connectivity, and Fig. 5 is clear evidence that the crystallinity does indeed spread from one layer to the next. 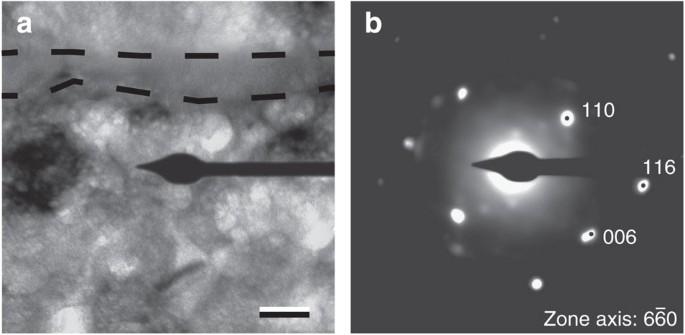Figure 5: TEM cross-section showing continuity of crystallinity across one organic layer. A trilayer of calorg/organics/calorgwas ion-beam milled to expose a cross-sectional surface. (a) TEM imaging (scale bar, 20 nm) and (b) electron diffraction reveals that pseudo-single crystallinity is maintained across this porous organic layer (bounded by the dashed lines ina). Figure 5: TEM cross-section showing continuity of crystallinity across one organic layer. A trilayer of cal org /organics/cal org was ion-beam milled to expose a cross-sectional surface. ( a ) TEM imaging (scale bar, 20 nm) and ( b ) electron diffraction reveals that pseudo-single crystallinity is maintained across this porous organic layer (bounded by the dashed lines in a ). Full size image These experiments were repeated along the organic interface, consistently showing that crystallinity was propagated from one cal org tablet to the next across the organic film. The crystal orientation was seen to change occasionally during the scan, but the lateral boundaries between adjacent tables could not be resolved in the TEM cross-sections. Single-crystal diffraction of a small-particle assembly The granular nature seen in Fig. 5a stems from the aggregation of polymer-induced liquid precursor droplets, which later crystallize into the tablets. The ED image in Fig. 5b reveals that this agglomeration of calcite nanoparticles diffracts as a single crystal, similarly to biogenic nacre. This seemingly paradoxical observation is common in biominerals, and is indicative of the oriented attachment of granular building blocks during calcium carbonate precipitation and crystallization under biological (or biomimetic) conditions. This is a result of the amorphous precursor, which forms nanoscale hydrated droplets that join to form an amorphous network, and later crystallize via a single nucleation event, or propagate the crystallinity of a crystal substrate. This is well documented for biological [32] , [33] , [34] , [35] , [36] , [37] and artificial [12] , [26] , [28] , [38] systems and thus further emphasizes the biomimetic nature of our artificial nacre. We present a route to artificial nacre, which resembles the biogenic material in terms of the detailed synthesis route, its structure as well as in its mechanical and optical properties. By carefully mimicking the steps in a cyclical deposition protocol, an organic-rich calcite mutlilayer stack that approximates biological nacre in all essential points was formed. These consist of (1) a 5–35-μm-sized polycrystalline cal org structure organized in 400-nm-thick plates that are (2) interconnected via the holes in the PVP layers, which ensures crystal continuity. (3) The composite structure gives rise to nacre-like enhanced toughness. (4) The good control over the layer periodicity reproduces nacre's iridescence. The close replication of nacre allows to test each of the biological steps, elucidating for example the interplay of organic pore structure and crystal domain size. Technologically, this biomimetic process heralds the manufacture of tough surface coatings from cheap base materials made by low temperature sustainable methods. Manufacture of artificial nacre PVP ( M n =60 kg mol −1 ), PAA ( M n =1.8 kg mol −1 ), PAA sodium salt (PAA–Na, M n =5 kg mol −1 ) and ammonium carbonate were bought from Sigma and used as received. Glass slides were cleaned by immersion in freshly prepared piranha solution (concentrated H 2 SO 4 :H 2 O 2 3:1 by weight) for 1 h at 100 °C followed by rinsing with 18.2 MΩ cm water. The substrates were coated with a continuous PVP film by spin coating from a 1% solution in ethanol at 3,000 r.p.m. for 1 min. This layer was crosslinked under 254 nm UV light for 5 min. Carboxyl functionalization was achieved by dipping in a 10 wt/v% PAA solution for 1 min followed by thorough rinsing in water. Samples were placed in a gas-permeable silicone beaker, secured against the side wall. The beaker was filled with 250 μl of PAA–Na stock solution (20 wt/v%) and 50 ml of a fresh aqueous solution of 16 mM CaCl 2 and 80 mM MgCl 2 . The beaker was placed in a 1 l sealed desiccator with 6 g of freshly crushed ammonium carbonate and left for 2 h at room temperature. ACC was deposited via hydrated Ca 2+ /Mg 2+ /PAA ion clusters, which coalesce to form a smooth film. The samples were removed, rinsed in pure water and dried in a nitrogen stream. Layer-by-layer deposition was carried out by sequentially immersing samples in a 100 ml 1 mg ml −1 PAA methanol solution for 2 min, followed by rinsing in two pure methanol solutions for 1 min each, then in a 100 ml 1 mg ml −1 PVP methanol solution followed by the same rinsing cycle. Using a Janome JR2400N robot, this two-step process was repeated 10–30 times to deposit a PAA/PVP layer with a well-defined film thickness. Samples were then placed in a pH 10 NaOH solution for 5 min. PAA dissolves out from the film during the first minute, followed by PVP dewetting into a porous membrane [21] . The films were rinsed in pure water for a further 5 min before the UV and PAA treatment and continued CaCO 3 growth as described above. The ACC film was finally crystallized by placing dry multilayers in the same desiccator with 10 ml of warm water for 6 h, causing a humidity of >95%. This gave rise to Mg and PAA-containing single crystal calcite. Note that in natural nacre aragonite forms from a similar Ca 2+ :Mg 2+ ratio in water. ACC-mediated aragonite growth has, however, not been replicated in vitro . This whole process forms a single bilayer and is repeated to form the artificial nacre. Sample characterization The biogenic and artificial nacre were imaged by optical microscopy with crossed polarisers. Reflection spectra were recorded using an angular resolved setup. The light from a incandescent source (Ocean Optics, with a wavelength-range of 230–2,000 nm) was incident on the sample via an optical fibre illuminating and area of 3 mm 2 . The illumination angle ranged between 15–75° with respect to the surface normal. The specularly reflected light was coupled into an optical fibre connected to an Ocean Optics QE65000 spectrometer. Thermogravimetric analysis was performed on a TA Instruments Q500 system, running from 25 to 900 °C under air flow. The angular resolution of the setup was ~1°. X-ray analysis was performed using a Bruker D8 diffractometer with a position-sensitive detector (LynxEye). A single CaCO 3 layer was grown on a silicon wafer with (510) crystal orientation, which has no diffraction peaks in the 2 θ region of interest. The diffraction pattern was compared with the spectra of calcite (PDF 83-0577) and dolomite (PDF 74-1687) crystals. For scanning electron microscopy, samples were fractured and sputter-coated with a 4-nm-thick Au/Pd layer. Scanning electron microscopy (SEM) imaging was performed on a LEO 1530 operating at 5 kV at a sample angle of 45°. A Veeco Dimension 3100 atomic force microscope was used in tapping mode to image the porous PVP layer. TEM-SAED to determine CaCO 3 crystallinity was carried out using a FEI Tecnai 20 on a CaCO 3 film on a holey carbon grid at 200 kV with a camera length of 890 mm. A 20 μm aperture was used for SAED of whole tablets, and 1 μm for cross-sections. Ion beam milling was performed on an FEI Philips Dualbeam Quanta 3D system. Mechanical measurements Nanoindentation tests were performed on a UBI 1 (now TI-700, Hysitron Inc., Minneapolis, MN) on a single crystal of aragonite, biogenic nacre sample, CaCO 3 film, replica and PVP. A Berkovich tip was employed for material property measurements in load control. A trapezoidal load profile was used, with 10 s loading, holding and unloading times. The peak load varied by sample to maintain indentation displacements in the range 30–150 nm (150, 250, 500 N for each material, respectively). Between 20 and 110 individual indentation tests were performed on each sample. The plain strain elastic modulus was calculated from the unloading stiffness via a calibrated tip-area function that was validated on fused silica and aluminium standard samples [39] . A cube-corner tip was used to investigate the fracture behaviour via nanoindentation. A triangular load profile was used with 2 s loading and unloading times. The peak load was 5 mN for aragonite and nacre samples and 1.5 mN for CaCO 3 and replica samples. Following cube-corner indentation, the residual indent was scanned in SPM mode at a contact force of 1.5–2 μN to ascertain whether cracking had occurred. Five individual indentation tests were scanned per sample. How to cite this article: Finnemore A, et al . Biomimetic layer-by-layer assembly of artificial nacre. Nat. Commun. 3:966 doi: 10.1038/ncomms1970 (2012).